Semiclassical Monte-Carlo approach for modelling non-adiabatic dynamics in extended molecules Modelling of non-adiabatic dynamics in extended molecular systems and solids is a next frontier of atomistic electronic structure theory. The underlying numerical algorithms should operate only with a few quantities (that can be efficiently obtained from quantum chemistry), provide a controlled approximation (which can be systematically improved) and capture important phenomena such as branching (multiple products), detailed balance and evolution of electronic coherences. Here we propose a new algorithm based on Monte-Carlo sampling of classical trajectories, which satisfies the above requirements and provides a general framework for existing surface hopping methods for non-adiabatic dynamics simulations. In particular, our algorithm can be viewed as a post-processing technique for analysing numerical results obtained from the conventional surface hopping approaches. Presented numerical tests for several model problems demonstrate efficiency and accuracy of the new method. Computational chemistry became a mature field able to address many problems of chemistry and materials science. Commonly, it numerically solves time-independent Schrödinger equation for electronic system of a molecule assuming the Born–Oppenheimer approximation, where electrons adjust instantaneously to the slower motion of the nuclei. Consequently, the (classical) nuclear positions enter as parameters to the electronic Hamiltonian , adiabatic many-body eigen functions and energies of electronic states [1] , [2] . The wavefunctions provide a complete characterization of the electronic system such as electronic density distribution, dipoles and optical responses. In addition, the adiabatic potential energy surfaces (PES) (generally -dimensional hypersurfaces in a space of all nuclear degrees of freedom , ) deliver information on the molecular energetics. Although complete mapping of molecular PES is impossible except for few-atom systems, efficient calculation of PES gradients (forces) and Hessians allows determination of global and local energy minima (optimal and meta-stable structures), location of transition states, energy barriers and so on. Development of adiabatic ab initio molecular dynamics made possible to propagate ‘on-the-fly’ Newton/Lagrange equations of motions for the nuclear degrees of freedom along the selected PES (ref. 3 ) The situation becomes more complex when the Born-Oppenheimer approximation becomes invalid, for example, when the neighbouring PESs become closely spaced (by about a few vibrational quanta) and the system attains a non-equilibrium state being excited to some superposition of excited states . This is the case of many important non-adiabatic dynamical phenomena such as non-radiative relaxation (for example, photoisomerization) [4] , [5] , intersystem crossing [6] , charge and energy transport in many technological applications (for example, photovoltaics, catalysis and energy storage) [7] , [8] , [9] , [10] and natural systems (for example, photosynthetic complexes) [11] , [12] . All these processes involve transitions between electronic states and the underlying electronic wavefunctions evolve in the space of multiple PESs. Many semiclassical approximations developed over the past decades are able to deal with this situation [13] , [14] , [15] , [16] , however, only a few methods can be effectively coupled with computational chemistry techniques enabling simulations of realistic molecular systems with ten-to-hundreds of atoms in size. Here most commonly used are mixed quantum-classical dynamics approaches, which generally operate with solutions of equations (1) and (2) [15] , [17] . The oldest approach, the Ehrenfest (or mean field) dynamics, propagates nuclei using an average force corresponding to the electronic subsystem being in a linear combination (superposition) of adiabatic states [18] . Surface hopping approaches (such as fewest switches surface hopping (FSSH) algorithm [19] ) typically average over a family of classical trajectories (equation (2)), where quantum transitions among states are allowed. The ab initio multiple spawning technique simultaneously solves nuclear dynamics (via evolution of frozen Gaussian wavepackets) and electronic structure problems [20] . The relative simplicity in these approaches comes at the expense of built-in severe approximations underlying inconsistencies between quantum and classical mechanics [17] . For example, proper treatment of electronic coherence evolution [10] , [12] remains challenging in all methods [21] , [17] , [16] . Nevertheless, important findings have been reported for large systems (such as organic molecules [20] , [5] , quantum dots [22] , [23] and carbon nanotubes [24] ) using the mixed quantum-classical techniques. A recent issue in the Journal of Chemical Physics [17] summarizes the current state of the field. In this paper, we propose a practical computational approach suitable for modelling non-adiabatic molecular dynamics in large molecular systems. Our semiclassical Monte-Carlo (SCMC) algorithm is based on a well-controlled physical approximation (that is, the Wentzel–Kramers–Brillouin approximation) and naturally couples to an arbitraty electronic structure theory (for example, density functional theory (DFT) and time-dependent DFT [1] , which became methods of choice for calculation of ground and excited state properties in extended systems, respectively). The quantum chemistry calculates only a few specific quantities for a given molecular geometry (input), namely, state energies , gradients (forces) and the first order non-adiabatic couplings (vectors NACR and scalars NACT ). The derivatives can be evaluated very efficiently using analytical approaches [25] , [26] . Unlike common surfaces hopping approaches, the SCMC is not ad hoc by its construction, and is able to account for the quantum interference effects between different photoinduced pathways [16] . Yet, its realization is based on the FSSH-like computational framework [19] , [17] : ‘on-the-fly’ propagation of equation (2) without prior knowledge of the PESs involved. The accumulated phase information characterizing each classical trajectory (for example, the action along the trajectory) is further used to perform ‘post-processing’ evaluation of multidimensional integrals using the Monte-Carlo technique [27] , [28] . Expression for the occupation probability of a certain state We consider a system with nuclei degrees of freedom and electronic levels. For simplicity, here we describe case; generalization to an arbitrary is straightforward and will be discussed later. We assume that initially the system occupies ’s electronic state ( ) with vibrational quantum state characterized by a product of Gaussians centred around classical (average) positions and momenta (see Supplementary Note 1 ). At a later time , the wavefunction of the full system can be written as , where coefficients are nuclei wavefunctions (or probability amplitudes) when the electronic subsystem occupies the ’th state. Herman [29] expressed the total probability for the electrons to occupy the ’th state, , via a semiclassical expansion in terms of the non-adiabatic couplings evaluated along the classical trajectories of nuclei [30] . Here we use its modified form (see Supplementary Notes 1,2 for a complete derivation using path integral formalism [31] ): where we have denoted and , and . Here , being the respective NACT. Equation (3) can be viewed as a (double) path integral (in the subspace of electronic levels, not nuclei!) over the paths corresponding to the sequences of hops at times and between electronic levels, starting in state and ending in state . Indices and denote the number of hops between electronic levels along a given trajectory. Phases are related to the classical actions of the nuclei as , where and classical momenta and coordinates of nuclei are taken at the endpoint time of a trajectory for which action in equation (4) is evaluated. Note that in equation (4) we have defined and . Functions are the overlap integrals of the gaussians corresponding to the wavefunctions of nuclei that evolved along different paths in the subspace of the electronic levels, that is, with different sequences of hops between these levels. Explicit expressions for and discussion of equation (3) are presented in the Supplementary Note 1 . Note that while trajectories of the nuclei entering equations (3 and 4) can be obtained by solving the classical equations of motion (for example, equation (2)), they should be supplemented by the boundary conditions connecting the nuclei velocities immediately before and after the hop. These boundary conditions, as suggested by Herman [29] , correspond to rescaling the velocity components along the NACR vector , so that the total energy of the system is conserved (see Supplementary Note 1 ). Sampling the integrand function with classical trajectories The main result of this study is formulation of the efficient SCMC algorithm that evaluates the integral series in equation (3) by Monte-Carlo method using a procedure similar to the traditional surface hopping approaches. However, unlike the latter, in the SCMC approach the classical trajectories are used to sample the integrand functions in equation (3). The algorithm consists of two (pre- and post-) processing steps. The first step is identical to the surface hopping schemes, for example, FSSH [19] . Namely, we propagate a swarm of classical trajectories according to equation (2) allowing the system to hop from the current PES to the other PES (or PESs in a general case). However, in our approach the hopping rate is arbitrary (that is, at each integration time step the system is allowed to hop to another PES with probability ). To preserve energy, as in the FSSH [17] , we assume that a hop occurs (at time and from ’th PES to the ’th PES) only if it is allowed by the energy balance condition, . Note, the hopping rates at the moments of hops and some phase information need to be retained along the classical trajectories as detailed below. In the second, post-processing step, the trajectories are sorted out into groups according to their final electronic states and the numbers of hops that occurred during their course. Each group represents a sample that is used to evaluate a corresponding integral in equation (3). That is, groups with and hops, both ending up on the ’th PES, correspond to the Monte-Carlo sample of the integrand function in the ’th integral (that is, the term with integrations over and integrations over in equation (3)), taken with respect to the probability distribution where (with and ) and are normalization coefficients, . Then, by multiplying and dividing the integrand function in the -fold integral in equation (3) by , the value of can be expressed as an average of function evaluated over the sample points and of the distribution function , where are the numbers of trajectories (that is, data points) with and hops. The function can be readily evaluated for a given pair of trajectories. Indeed, one can easily calculate phases and values of function for each trajectory, as well as the overlap integrals for the pair. The value of , on the other hand, is unknown as one does not know the values of the normalization constants . These constants, however, can be determined from the statistics of the stochastic process defined by the rates , that is, from the numbers of trajectories that finished at the ’th PES after hops. As hops are independent, one can readily evaluate the probability of such a trajectory. Rather straightforward combinatorial considerations (see Supplementary Note 2 for details) yield where . In the case of multiple PESs in this expression should be replaced by , that is, the escape rate to the other states. The integral in equation (7) can be found by a similar Monte-Carlo procedure. Indeed, introducing probability distribution , the same as in equation (5), one rewrites the rhs of equation (7) as an average taken with respect to the sample, , with . As the value of can be readily evaluated for each trajectory, the above expression can be used to calculate the probability , provided one knows . On the other hand, if and the total number of trajectories are both sufficiently large numbers, , then the normalization constants entering equations (5, 6) for evaluation of are Notably, the SCMC algorithm can be readily generalized to the case of an arbitrary number of the PESs. For , each term in the series in 1quation (3) must contain all possible transitions among levels, for both and hop paths; hence the integrals over and should be supplemented with the sums and over the intermediate PESs that system has hopped while travelling from the initial to final state. This forms distribution functions and averages over the corresponding samples including the discrete subspace of electronic levels together with the continuous space spanned over temporal positions of jumps. Application of the SCMC algorithm to Tully’s test suite Tully’s three model ‘chemical’ problems [19] involving a single nuclei degree of freedom and two coupled electronic levels, present a standard test suite for non-adiabatic molecular dynamics algorithms. Figures 1 , 2 , 3 demonstrate that a simple choice of hopping rate, , yields a very good agreement between the results obtained with the SCMC and the exact numerical results for all three model problems (for comparison, these figures also show the results obtained by the mean field (Ehrenfest) and FSSH methods). The figures display the scattering probabilities (for large times) as a function of initial momenta of the particle. In all three problems, the particle is localized initially on the lower PES with momentum directed towards the non-adiabatic region. The PES forms and the absolute values of the non-adiabatic couplings are shown in (a) of the figures; the details, such as the explicit form of the Hamiltonians and the initial wavefunction, are presented in Methods. In particular, qualitative failures of the Ehrenfest and FSSH methods are well recognized for model problem 3 (for example, see Fig. 3b ) [19] , [17] . Here, the SCMC essentially reproduces the exact result, which indicates the proper accounting for the quantum interference effects and dynamics of electronic coherences [21] , missing, for example, in the FSSH approach. 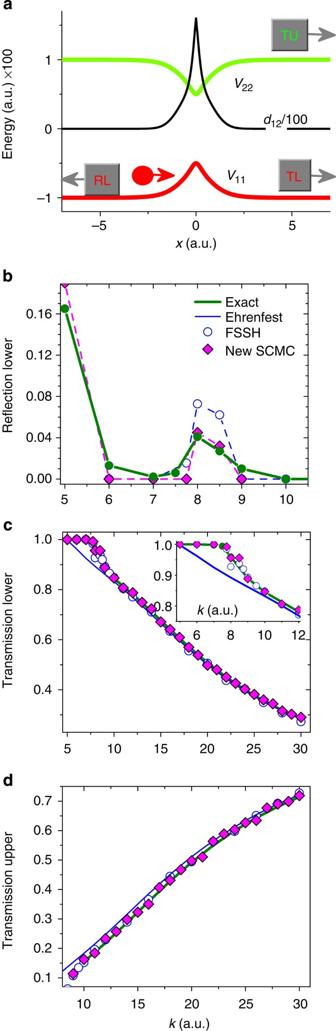Figure 1: Scattering probabilities for the test problem 1 (simple avoided crossing). (a) Shows energy levels and non-adiabatic coupling. (b–d) Display calculated scattering probabilities. Samples of 25,000 and 10,000 trajectories for each data point were used to compute the SCMC and FSSH results, respectively. Figure 1: Scattering probabilities for the test problem 1 (simple avoided crossing). ( a ) Shows energy levels and non-adiabatic coupling. ( b–d ) Display calculated scattering probabilities. Samples of 25,000 and 10,000 trajectories for each data point were used to compute the SCMC and FSSH results, respectively. 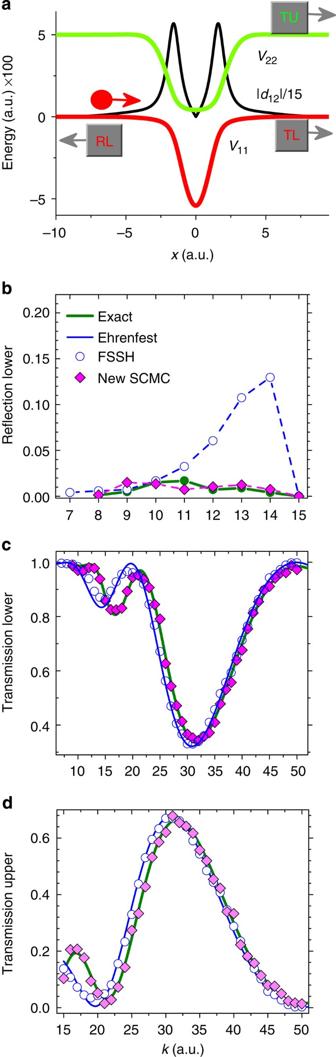Figure 2: Scattering probabilities for the test problem 2 (double avoided crossing). (a) Shows energy levels and non-adiabatic coupling. (b–d) Display calculated scattering probabilities. Samples of 75,000 and 10,000 trajectories for each data point were used to compute the SCMC and FSSH results, respectively. Full size image Figure 2: Scattering probabilities for the test problem 2 (double avoided crossing). ( a ) Shows energy levels and non-adiabatic coupling. ( b–d ) Display calculated scattering probabilities. Samples of 75,000 and 10,000 trajectories for each data point were used to compute the SCMC and FSSH results, respectively. 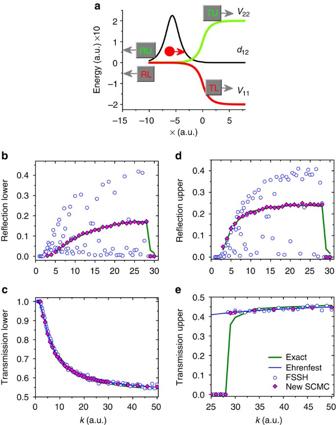Figure 3: Scattering probabilities for the test problem 3 (extended coupling with reflection). (a) Shows energy levels and non-adiabatic coupling. (b–e) Display calculated scattering probabilities. Samples of 25,000 and 10,000 trajectories for each data point were used to compute the SCMC and FSSH results, respectively. Full size image Figure 3: Scattering probabilities for the test problem 3 (extended coupling with reflection). ( a ) Shows energy levels and non-adiabatic coupling. ( b – e ) Display calculated scattering probabilities. Samples of 25,000 and 10,000 trajectories for each data point were used to compute the SCMC and FSSH results, respectively. Full size image Application of the SCMC algorithm to multidimensional problem Finally, application of the SCMC approach to the model multidimensional problems [32] , [33] , [34] represents an important test of numerical convergence in cases where nearby trajectories are diverging or converging. This may potentially result in large prefactors which off-set favourable numerical cost scaling of the present method with the number of vibrational degrees of freedom (see Discussion below). We use model 2D problem introduced in Shenvi et al . [34] , which involves two nuclear degrees of freedom and a rather non-trivial geometry of two PES ( Fig. 4a ) and the corresponding NACR vector field ( Fig. 4b ). This is a non-separable 2D problem providing a natural extension of 1D Tully problem 2 to the higher dimensions (see Methods for an explicit form of the Hamiltonian and the initial wavefunction). Subsequently, the exact solution (numerically tractable only for a moderate range of the initial wavepacket momentum, 15 k 45) displays significant so-called Stueckelberg oscillations [35] , which are also present in problem 2 ( Fig. 2c ). These oscillations appear when the probability amplitudes evolving along two potential curves interfere, and render the conventional methods to be rather inaccurate [34] (for example, Fig. 4d ). Moreover, in problem 4, the size of the non-adiabatic region for this problem is comparable to the width of the wavepacket, which puts the underlying semiclassical approximation to a stringent test. In spite these challenges, our numerical SCMC results agree well with the exact data ( Fig. 4d ). The observed deviations are related to the simple Gaussian approximation for the shape of the wavepacket used in the algorithm, which was assumed to correspond to that for a free particle. The error can be reduced by computing the time-dependence of the wavepacket’s width ‘on-the-fly’ for each trajectory; a particularly convenient way to do it has been introduced by Heller [36] . Such refinement would, however, lead to the necessity to evaluate the second derivatives of (with respect to ), which can possibly increase the numerical cost of the underlying electronic structure calculations when applied to realistic molecular systems but not in the SCMC evaluation itself. Finally, we point out, that the numerical cost of our algorithm is practically invariant with respect to the number of the nuclear degrees of freedom, as exemplified by the test problem 4. Indeed, in both problems 2 and 4 we observe the same convergence rate despite the latter one has an extra spatial (nuclear) degree of freedom. This fact is not surprising: the dynamics of the nuclei between the hops is fully deterministic and the sampling is done in the space of the electronic states only. 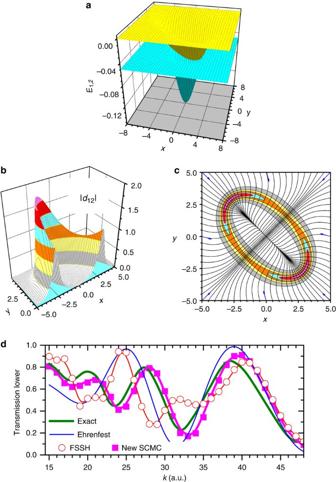Figure 4: Numerical results for the two-dimensional test problem 4. (a–c) Show forms of two PESs and the corresponding NACR vector field, respectively. (d) Display calculated scattering probabilities for the system to occupy the second (lower) PES. Samples of 75,000 and 10,000 trajectories for each data point were used to compute the SCMC and FSSH results, respectively. Figure 4: Numerical results for the two-dimensional test problem 4. ( a – c ) Show forms of two PESs and the corresponding NACR vector field, respectively. ( d ) Display calculated scattering probabilities for the system to occupy the second (lower) PES. Samples of 75,000 and 10,000 trajectories for each data point were used to compute the SCMC and FSSH results, respectively. Full size image After formulating the SCMC algorithm and its numerical tests, here we discuss the essential features, advantages and the future outlook of this approach. First, Scalability: Our method of Monte-Carlo sampling is invariant with respect to the number of vibrational degrees of freedom ( ). In contrast, in the previous proposals (for example, Herman [37] ) using semiclassical expressions similar to equation (3) to model non-adiabatic dynamics, the computational complexity scales (presumably) exponentially with or results in a poor convergence [38] . In terms of electronic states , formally, in the SCMC there is a significant expansion of the sampling space (by a factor for each term in equation (3)). This reflects an increase of all possible products during dynamics in the multilevel system. However, in the realistic molecular systems, typically there are only a few photoinduced pathways heavily dominating the excited state dynamics. These pathways are well identified even on the first step, when conducting hopping dynamics simulation. Consequently, we expect that most paths (in the subspace of electronic levels) can be divided into relatively few groups with common sequences of hops that represent samples of the most relevant integrals in equation (3) (see an extension to the case of arbitrary in the Supplementary Notes 1 and 2 ). Second, Convergence and hopping rates: Although the SCMC approach formally allows for arbitrary hopping rates, a poor choice may result in an unreasonably high computational cost for the evaluation of the integrals in equation (3). We note that the total unnormilized probability for all products (equal to one in the limit of infinite sample, as confirmed by the numerical tests) provides a natural criterion of the SCMC convergence. Compared with the FSSH, the SCMC approach requires larger sample of trajectories in order to achieve comparable to FSSH convergence ( Figs 1 , 2 , 3 , 4 ). Partially, this is due to interference effects between trajectories containing the phase information. Moreover, our choice of the hopping rates used is far from optimal. Indeed, while such choice of properly accounts for an amplitude of the integrand function, it is clearly ‘unaware’ of its oscillatory behaviour leading to significant errors in small samples. To improve the sampling efficiency, [38] one might use that increases in the regions with rapidly varying , and so on. Other possibilities include use of the stationary state Monte-Carlo [39] , [40] , [41] and analytical continuation method [42] applied in evaluation of conventional path integrals. In general, the hopping rate choice is related to the optimization of an important sampling function explored in many other Monte-Carlo schemes [27] , [43] . Third, Thermal noise and bath effects are commonly included into simulations to model molecular environment [44] . Although equations (2) and (3) do not account for these phenomena, inclusion of the thermal effects will not change significantly the outlined sampling protocol [38] . However, it will lead to the diffusion of the nuclei and, therefore, will affect the overlap integrals and the simulation results at both quantitative and qualitative levels. In summary, we have proposed a new computational paradigm to model non-adiabatic dynamics based on a hybrid of semiclassical approximation and surface hopping method invoking Monte-Carlo sampling of multidimensional integrals (equation (3)). Although our findings and numerical tests are very encouraging, most importantly, we believe that this work opens a broad field of future studies on how to improve the proposed protocol (for example, how to refine the sampling efficiency), which is closely connected to other formally unrelated areas of computer and physical sciences utilizing complex Monte-Carlo schemes. For example, one may start asking questions on how to define the optimal important sampling function [38] (here hopping rate) to probe a very specific photoinduced pathway (which potentially may be a rare event). We expect, that the proposed method to become a standard tool that will be used to address a variety of problems in photoinduced molecular dynamics (such as coherent excited state dynamics [10] , [12] ) and will complement the existing approaches (for example, Ehrenfest and FSSH). Numerical test The Hamiltonian operator for all four test problems takes the form where is a nuclear coordinate and matrix describes two coupled electronic PES. The wavefunction of the system is thus a two-component vector . The potential energy matrix (that is, in equation (9)) has non-adiabatic coupling vector , which is nonzero in the vicinity of the origin ( ). In all test problems, the mass of the particle is taken close to proton's mass, The first three problems are one-dimensional, that is, . The first problem corresponds to a single avoided level crossing (see the energy levels, that is, the eigenstates of , in Fig. 1a ) the coefficients of the matrix are given by while for the second problem, a double avoided level crossing ( Fig. 2a ) the coefficients are given by In the third, the so-called ‘extended coupling with reflection’ problem ( Fig. 3a ), the coefficients of the potential energy matrix are In all three problems the particle starts with a wavefunction where is negative and relatively large in absolute value (we take ) and , being the initial momentum (here and in the following all quantities are measured in atomic units). All the parameters are the same as in Tully [19] . The wavepacket, initially at the lower energy level (equation (10)), propagates toward the region with nonzero adiabatic coupling (that is, ) and scatters off the effective potential, thus forming the transmitted and the reflected wavepackets on lower or upper PESs, schematically shown in (a) of Figs 1 , 2 , 3 . We evaluate numerically the probabilities of forward and backward scattering (that is, transmission and reflection probabilities) into the two levels at (for transmission) and at (for reflection) at sufficiently large times (that is, at ). These probabilities are evaluated as where subscript labels the electronic level ( ), the superscripts correspond to transmission and reflection, and is obtained by solving the time-dependent Schrödinger equation with the Hamiltonian (equation (9)) subject to the initial condition (equation (13)). Problem 4 is two dimensional ( Fig. 4a ), that is, , with all parameters taken from Shenvi et al . [34] : Following Shenvi et al . [34] , the initial wavefunction is given by where and . Figure 4d shows the full probability of the system to occupy the second (lower) PES at , where is the adiabatic eigenstate corresponding to the second PES. In equations (10, 11, 12, 13, 14, 15), the energy and the distance are measured in atomic units ( ). How to cite this article: Tretiak S. et al . Semiclassical Monte-Carlo approach for modelling non-adiabatic dynamics in extended molecules. Nat. Commun. 4:2144 doi: 10.1038/ncomms3144 (2013).